Giant non-reciprocity at the subwavelength scale using angular momentum-biased metamaterials Breaking time-reversal symmetry enables the realization of non-reciprocal devices, such as isolators and circulators, of fundamental importance in microwave and photonic communication systems. This effect is almost exclusively achieved today through magneto-optical phenomena, which are incompatible with integrated technology because of the required large magnetic bias. However, this is not the only option to break reciprocity. The Onsager–Casimir principle states that any odd vector under time reversal, such as electric current and linear momentum, can also produce a non-reciprocal response. These recently analysed alternatives typically work over a limited portion of the electromagnetic spectrum and/or are often characterized by weak effects, requiring large volumes of operation. Here we show that these limitations may be overcome by angular momentum-biased metamaterials, in which a properly tailored spatiotemporal modulation is azimuthally applied to subwavelength Fano-resonant inclusions, producing largely enhanced non-reciprocal response at the subwavelength scale, in principle applicable from radio to optical frequencies. Non-reciprocity in ferromagnetic materials originates from the unidirectional precession of electron spins [1] or the Zeeman splitting of atomic orbitals [2] in the presence of a static magnetic bias. There is a large interest in mimicking this effect in artificial materials without requiring applied magnetic fields, but instead relying on bias with other odd vectors under time reversal in compliance with the general principle of microscopic reversibility [3] . Such possibility would relax the current requirements of large magnetic biasing devices in non-reciprocal components, with the potential of revolutionizing the microwave and photonic component industry. Kodera et al . [4] , for instance, present a non-reciprocal metamaterial composed of transistor-loaded ring resonators, where suitably designed active loads, biased with direct electric current, can suppress one of the two azimuthally propagating eigenstates, producing a unidirectionally rotating magnetic moment functionally equivalent to ferromagnetic effects. Although this approach can be used to realize some non-reciprocal components [5] , [6] , it is limited to microwave and millimetre-wave frequencies, where transistors are available, and it involves significant power consumption in the transistors’ biasing network. Another transistor-based, current-biased non-reciprocal metamaterial was proposed in ref. 7 , consisting of cross-polarized dipoles interconnected to each other via transistors to achieve symmetry breaking and microwave Faraday rotation, with similar limitations. [8] , [9] , [10] , [11] , [12] , [13] Refs 8–13 present a different class of non-reciprocal components. In this case, biasing is provided by the linear momentum vector imparted by longitudinal spatiotemporal modulation suitably tailored to break time-reversal symmetry. This concept can provide optical isolation by means of direct or indirect interband photonic transitions in spatiotemporally modulated waveguides. Direct transitions [10] can be described as the photonic equivalent of the Aharonov–Bohm effect, whereas indirect transitions [8] occur in the presence of a traveling wave modulation breaking space-inversion and time-reversal symmetries. The proposed devices can be broadband but their size is determined by the coherence length of the transitions, which, for reasonable modulation amplitudes, is several wavelengths, making these devices rather bulky. Nonlinearities have also been proposed to induce non-reciprocity [14] , [15] , [16] , [17] , [18] but the operation of the resulting devices is limited to specific ranges of input power. All these solutions rely on inherently weak effects, requiring large volumes, and are therefore not necessarily preferable to conventional solutions based on magneto-optical effects. The field of optical metamaterials has also offered opportunities for boosting the non-reciprocal response of magneto-optical materials by means of large field enhancement and localization. Two recent examples are plasmonic-enhanced Faraday rotation [19] and isolation enabled by parity-time symmetry [20] . In the following, we suitably combine the strong wave–matter interaction of resonant metamaterial inclusions with the non-reciprocal properties of a new form of spatiotemporal modulation aimed at imparting a bias based on the angular momentum vector. We show that this combination can induce giant non-reciprocal response at the subwavelength scale, leading to the introduction of a new type of linear, non-reciprocal phenomenon based on angular momentum-biased metamaterials, which can overcome the limitations of the aforementioned approaches with potentially groundbreaking applications in microwave and nanophotonic integrated systems. Principle of angular momentum-biased metamaterials The simplest constituent inclusion suited to form the proposed metamaterial is a ring resonator with an azimuthal spatiotemporal permittivity modulation Δ ε ( φ , t )=Δ ε m cos ( ω m t − L m φ ), as depicted in Fig. 1a , where φ is the azimuthal coordinate in a cylindrical reference system co-centred with the inclusion and L m is the modulation orbital angular momentum. In absence of modulation, Δ ε m =0, the ring supports degenerate counter-propagating resonant states with azimuthal dependence e iφ , resonating when the ring circumference is times the guided wavelength, which implies that, for the fundamental |±1 states used herein, the ring dimensions are smaller than the wavelength. The resonant size can be further reduced by adding capacitances along the loop, as in split-ring resonator designs [21] . As it will be shown shortly, introducing the aforementioned spatiotemporal azimuthal modulation lifts the degeneracy between the |±1 states and produces non-reciprocity, an effect that can be interpreted as the metamaterial analogue of a static magnetic bias removing the degeneracy between atomic states of opposite orbital angular momenta in magnetic materials. 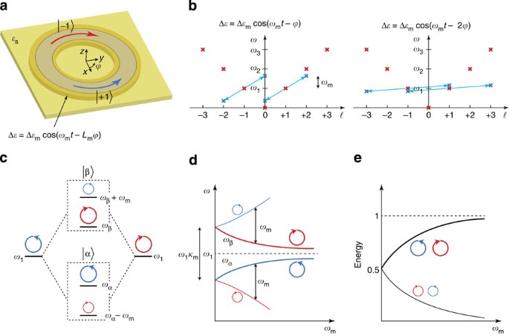Figure 1: Principle of non-reciprocal angular momentum-biased metamaterials. (a) Azimuthally symmetric ring resonator with a spatiotemporal modulation of permittivity. The modulation follows the form of an azimuthally propagating wave in the +φdirection. In the absence of modulation, the resonator supports two degenerate counter-propagating states |±1. The applied modulation lifts the degeneracy and produces non-reciprocity. (b) Transformation of the |±1states in the frequency and angular momentum plane forLm=1 (left) andLm=2 (right). Red crosses: states of the unmodulated ring. Blue crosses: intermodulation products. (c) Frequency diagram of the ring eigenstates without (left and right columns) and with (middle column) modulation forLm=2. The states of the modulated ring are hybridizations of the |±1states. Each hybrid state consists of a dominant (thick line) and a secondary (thin line) sub-state. (d) Sub-state eigenfrequencies versus the modulation frequency forLm=2. (e) Sub-state energies versus the modulation frequency forLm=2. Figure 1: Principle of non-reciprocal angular momentum-biased metamaterials. ( a ) Azimuthally symmetric ring resonator with a spatiotemporal modulation of permittivity. The modulation follows the form of an azimuthally propagating wave in the + φ direction. In the absence of modulation, the resonator supports two degenerate counter-propagating states |±1 . The applied modulation lifts the degeneracy and produces non-reciprocity. ( b ) Transformation of the |±1 states in the frequency and angular momentum plane for L m =1 (left) and L m =2 (right). Red crosses: states of the unmodulated ring. Blue crosses: intermodulation products. ( c ) Frequency diagram of the ring eigenstates without (left and right columns) and with (middle column) modulation for L m =2. The states of the modulated ring are hybridizations of the |±1 states. Each hybrid state consists of a dominant (thick line) and a secondary (thin line) sub-state. ( d ) Sub-state eigenfrequencies versus the modulation frequency for L m =2. ( e ) Sub-state energies versus the modulation frequency for L m =2. Full size image The proposed permittivity modulation is a type of amplitude modulation and, as such, it results in the generation of two intermodulation products and for each state | k . If any of them overlaps in frequency with another state , resonant coupling between the | k and state occurs, significantly affecting both resonances. As our goal is to lift the degeneracy between |±1 states, L m =1 and ω m = ω 2 − ω 1 might appear the most reasonable choice, so that the |+1 state gets resonantly coupled to the |+2 state, whereas no coupling occurs for the |−1 state, as illustrated in Fig. 1b , left panel. However, ω 2 is usually close to 2 ω 1 and, as a result, ω m should be close to ω 1 , which may be challenging to achieve especially at terahertz and optical frequencies. For L m =2, in contrast, the states |±1 resonantly couple to each other for ω m =0, as illustrated in Fig. 1b , right panel. For ω m identically zero, the structure is obviously reciprocal but any small departure from zero can break reciprocity and, no matter how large ω 1 is, strong non-reciprocal response may be obtained by properly choosing Δε m and the resonator Q -factor, as will be discussed in more detail in the following. This concept may be analysed using coupled-mode theory as in ref. 22 : the amplitudes a 1 of the |±1 states satisfy the equations (see Methods for details) where is the coupling coefficient between the |±1 states, with S t being the resonator cross-section and E t1 the corresponding normalized electric field distribution. For homogeneous resonators (Δ ε m and ε uniform, where ε is the background permittivity), κ m =Δ ε m /2 ε . The solution of equation (1) provides the eigenstates of the modulated ring (see Supplementary Note 1 for details): where ω α = ω 1 −Δ ω /2, ω β = ω 1 +Δ ω /2 and Δ ω = − ω m . This solution may be extended to take into account the presence of loss and coupling with the excitation signals, as discussed in the Methods section. The states |α and |β are hybridizations of the non-modulated ring states |+1 and |−1 , which are generally characterized by different frequencies and amplitudes, as illustrated in Fig. 1c . In the absence of modulation ( ω m =0), the sub-states |±1 of each hybrid state share the same frequency and energy, as shown in Fig. 1d,e , respectively, and the system is reciprocal as expected. However, when modulation is introduced ( ω m ≠0), the sub-states split ( Fig. 1d ) and non-reciprocity arises. This splitting follows from the simultaneous spatial and temporal nature of the proposed modulation, generating the states and from | k e − iωt ( Fig. 1b ). Therefore, if the sub-state |+1 exists at frequency ω , the sub-state |−1 can only exist at frequency ω − ω m . For ω m ≠0, the energy is unevenly distributed between sub-states ( Fig. 1e ) with the unbalance increasing with ω m . The dominant sub-states for |α and |β are |+1 and |−1 , respectively, as indicated in Fig. 1c–e with thick lines. The amount of non-reciprocity is determined by the minimum distance between sub-states of opposite handedness Δ ω min =min{ ω m , ω β − ω α =Δ ω } and by the resonance width ω 1 / Q , where Q is the resonance quality factor, corresponding to the inverse of the fractional bandwidth. In practical devices such as polarization rotators and circulators, which are based on interference between states, Δ ω min and ω 1 / Q must be of the same order [23] . In the Supplementary Note 1 , we prove that Δ ω min ≤Δ ω 1 κ m / , with the maximum value holding for ω m =Δ ω = ω 1 κ m / . Therefore, Qκ m = , consistently with the expectation that a lower Q resonator requires a higher κ m and subsequently a higher Δ ε m . Microwave Fano-resonant metasurface Consider now a spatiotemporally modulated metasurface consisting of periodically arranged pairs of broadside-parallel metallic rings patterned on both sides of a thin dielectric layer, as in Fig. 2a . Permittivity modulation is effectively obtained by loading the rings with time-variable capacitors Δ C n =Δ C m cos ( ω m t −2 φ n ) at the azimuthal positions φ n = nπ /4, where n =0…7, which is equivalent to applying a continuous capacitance modulation Δ C =(4Δ C m / π )cos( ω m t −2 φ ), as shown in the Methods section. It is noteworthy that the modulation amplitude 4Δ C m / π is the average of the localized capacitance Δ C m over the discretization period π /4, as it may be intuitively expected. A possible practical implementation of this capacitance modulation is illustrated in Fig. 2b : it consists of a varactor, as its core element, a direct current-biasing source, an alternating current modulation source with frequency ω m and appropriate filters that minimize the interference between the ring and the biasing network (see Supplementary Note 2 for details). Such a circuit may be easily integrated into the ring substrate within conventional printed circuit technology. Further, as varactors and filters are low-loss components, the overall power consumption is expected to be very low (in principle zero for ideally lossless circuit elements). 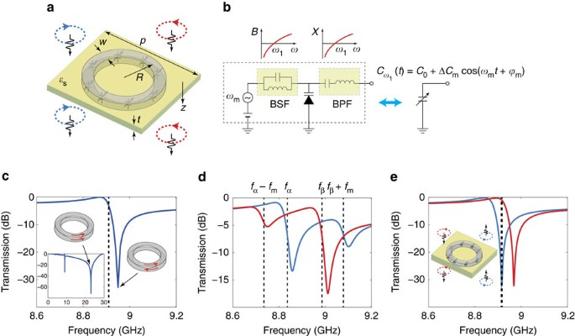Figure 2: Angular momentum-biased metasurface. (a) Constituent inclusion of the metasurface: a ring-pair resonator periodically loaded with time-variable capacitors. (b) Practical implementation of the time-variable capacitors: a band-stop filter (BSF) and a band-pass filter (BPF) are used to minimize the leakage of ring and modulation signals to the biasing network and to the ring, respectively. The two filters are designed to have zero susceptance and zero reactance at the ring resonanceω1, respectively. (c) Transmission through the unmodulated metasurface. A Fano-type resonance is supported at 8.9 GHz, resulting from the interference of a high-Qmagnetic (anti-parallel currents) resonance and a low-Qelectric (parallel currents) one. (d) Transmission across the metasurface in the +zdirection with ΔCm=0.02 pF andfm=0.1 GHz. Blue line: RHCP incidence. Red line: LHCP incidence. (e) Same as indbut forfm=0.5 GHz. If the propagation direction is reversed (from +zto −z), the RHCP and LHCP curves flip. At 8.91 GHz (dashed line), the metamaterial operates as an electromagnetic diode for CP waves; RHCP and LHCP waves can only propagate along the −zand +zdirections, respectively. The geometrical parameters of the structure areR=2 mm,w=1 mm,t=0.4 mm,εs=9 andp=3.4R. Figure 2: Angular momentum-biased metasurface. ( a ) Constituent inclusion of the metasurface: a ring-pair resonator periodically loaded with time-variable capacitors. ( b ) Practical implementation of the time-variable capacitors: a band-stop filter (BSF) and a band-pass filter (BPF) are used to minimize the leakage of ring and modulation signals to the biasing network and to the ring, respectively. The two filters are designed to have zero susceptance and zero reactance at the ring resonance ω 1 , respectively. ( c ) Transmission through the unmodulated metasurface. A Fano-type resonance is supported at 8.9 GHz, resulting from the interference of a high- Q magnetic (anti-parallel currents) resonance and a low- Q electric (parallel currents) one. ( d ) Transmission across the metasurface in the + z direction with Δ C m =0.02 pF and f m =0.1 GHz. Blue line: RHCP incidence. Red line: LHCP incidence. ( e ) Same as in d but for f m =0.5 GHz. If the propagation direction is reversed (from + z to − z ), the RHCP and LHCP curves flip. At 8.91 GHz (dashed line), the metamaterial operates as an electromagnetic diode for CP waves; RHCP and LHCP waves can only propagate along the − z and + z directions, respectively. The geometrical parameters of the structure are R =2 mm, w =1 mm, t =0.4 mm, ε s =9 and p =3.4 R . Full size image In the absence of modulation, the metasurface exhibits two resonances, shown in the inset of Fig. 2c , a low- Q ‘bright’ mode at 23 GHz with parallel currents induced in the two rings and a coupled high- Q ‘dark’ mode at 9 GHz with anti-parallel currents. Suitable coupling between these two modes results in a peculiar Fano-resonant response [24] , [25] at 8.9 GHz, with a sharp transition from full to no transmission ( Fig. 2c ). This response is ideal for our purpose, as its sharp frequency response relaxes the requirements on the modulation capacitance and, at the same time, leads to strong non-reciprocal effects because of the associated anti-parallel currents in the rings, maximizing the excitation of the modulation capacitors. Figure 2d shows the transmission of circularly polarized (CP) waves through the metasurface (along + z ) for Δ C m =0.02 pF and f m =100 MHz. The chosen value of Δ C m corresponds to an effective capacitance modulation of 0.026 pF rad −1 , which, considering the ring-pair capacitance 0.48 pF rad −1 , leads to κ m =0.027. This yields ω 1 κ m 0.24 GHz, which is enough for a clear separation between |α and |β states, consistent with the discussion in the previous subsection. Small variations of Δ C m that may occur in practice can be easily compensated by adjusting ω m as long as the |α and |β states are distinguishable. As expected, the response is different for right-handed CP (RHCP) and left-handed CP (LHCP) excitations, and in each case two resonant dips are observed, with the stronger one resulting from coupling with the state whose dominant sub-state is of the same handedness as the incident wave. RHCP incident waves strongly couple to |α at frequency f α , whereas LHCP waves strongly couple to |β at f β . The weaker resonant dips correspond to the secondary sub-states at f β + f m (RHCP excitation, substate |+1 of |β ) and f α − f m (LHCP waves, |−1 of |α ). If the structure is excited from − z , the transmission curves of Fig. 2d switch handedness as the incident wave feels opposite modulation spin, a clear demonstration of non-reciprocity. This polarization transmission asymmetry can be exploited to realize, for instance, a CP isolator by placing the transmission null of one polarization at the same frequency as the transmission peak of the other polarization. This condition is fulfilled for f m =0.5 GHz, as shown in Fig. 2e ; at 8.91 GHz RHCP and LHCP waves can penetrate the metasurface only from − z and + z , respectively. This operation may be the basis of different types of polarization-dependent microwave isolators. Another important non-reciprocal effect, common in ferromagnetic materials, is Faraday rotation, that is, the non-reciprocal rotation of the polarization plane of a wave, as it propagates through the material. The rotation is opposite for opposite propagation directions, as it is determined by the (fixed) bias direction. We can achieve the same effect in the proposed spatiotemporally modulated metasurface, as shown in Fig. 3a , which plots the polarization rotation angle θ for different f m and Δ C m =0.02 pF. As the modulation frequency increases, θ increases and the bandwidth decreases. The bandwidth reduction is clearly because of the decrease of Δ ω as f m increases, but the monotonic increase of θ may seem contradictory with the fact that the separation between states, which determines the amount of non-reciprocity, is actually reduced as f m increases. As shown in Fig. 3b , this peculiar monotonic increase of θ results from the fact that at resonance, for f m >0.5 GHz, the transmission coefficient for x -polarized waves T xx decreases faster than the transmission coefficient of x - to y -polarized waves T yx , so that T yx / T xx , which is proportional to θ , actually increases. For f m =0.5 GHz, T yx is maximum and θ =60°, corresponding to a giant rotation of 6,000° per free-space wavelength, without the need of any magnetic bias. In Fig. 3c , we show the ellipticity angle χ at the output for linearly polarized inputs. It is easy to see that this angle is zero at the frequency of maximum θ , implying that the transmitted field is linearly polarized, making the proposed metasurface particularly exciting for applications requiring non-reciprocal linear polarization rotation. 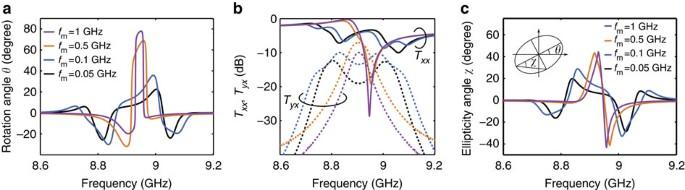Figure 3: Faraday rotation for the angular momentum-biased metasurface. (a) Rotation angle. (b) Transmission coefficient fromx- tox-polarized waves,Txx, and fromx- toy-polarized waves,Tyx. (c) Ellipticity angle: at the frequency of maximum rotation the ellipticity angle is zero, corresponding to ideal Faraday rotation. All the results were derived for the same ring parameters as inFig. 2. Figure 3: Faraday rotation for the angular momentum-biased metasurface. ( a ) Rotation angle. ( b ) Transmission coefficient from x - to x -polarized waves, T xx , and from x - to y -polarized waves, T yx . ( c ) Ellipticity angle: at the frequency of maximum rotation the ellipticity angle is zero, corresponding to ideal Faraday rotation. All the results were derived for the same ring parameters as in Fig. 2 . Full size image Optical isolator As pointed out above, the proposed scheme of spatiotemporal modulation with L m =2 poses no restriction on the modulation frequency, opening the possibility to apply the proposed concept to optical frequencies. As a proof of concept, an optical isolator based on a spatiotemporally modulated channel-drop filter is presented in Fig. 4 , with the design details provided in the caption. Without modulation, the power entering the structure through the channel waveguide (right-hand-side waveguide) from either port 1 or 2 couples to the right- or left-handed ring resonance, respectively, creating a transmission dip at resonance ( Fig. 4a ). Splitting the ring resonances with proper azimuthal spatiotemporal modulation moves the transmission dips to different frequencies for opposite propagation directions, thus creating non-reciprocity. The isolator can be realized on silicon (Si), which exhibits the strongest electro-optic effect observed to date, with typical values around Δ ε m =5 × 10 −4 ε s , where ε s is its permittivity, leading to κ m 2.5 × 10 −4 (refs 26 , 27 ). Such permittivity modulation can be obtained using pin diodes, as analytically described in refs 9 , 26 , 27 . According to our bandwidth criterion QC m = , a Q -factor ~7,000 would be sufficient for adequate separation of the |α and |β states. Such level of Q -factor is common in Si-photonics integrated systems, and in the design of Fig. 4a it is achieved using the 11th azimuthal resonance of the ring. Although the theory above was derived for the |±1 states, it can be easily extended to any pair of states by substituting L m =2 with L m =2 . Therefore, L m =22 was used in the design of Fig. 4 , which may be achieved by uniformly integrating 88 pin diodes along the ring perimeter, leading to a separation of 65 nm between consecutive diodes. It should be noted that this design has not been optimized, and our theory indicates that a significantly lower number of pin diodes may still be sufficient to achieve a similar effect in optimized geometries. 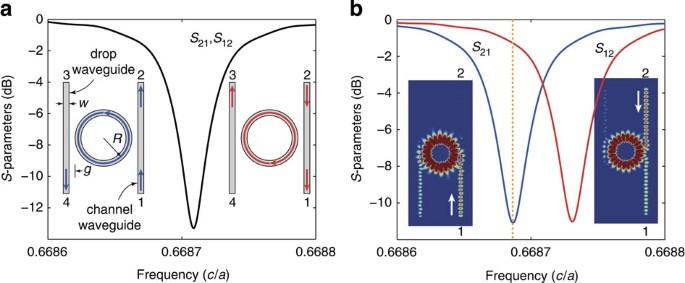Figure 4: Angular momentum-biased optical isolator based on a channel-drop filter. (a) Reciprocal transmission versus frequency of a conventional channel-drop filter. Waves entering from ports 1 and 2 couple to the right- and left-handed resonances of the ring, as illustrated in the left and right insets, respectively, creating a transmission dip at the ring resonance. (b) Non-reciprocal transmission versus frequency when spatiotemporal modulation is applied to the ring. The insets show the electric field amplitude distribution at the frequency indicated by the dashed line for excitation from port 1 (left) or 2 (right). The geometrical parameters of the structure areR=0.88a,w=0.2aandg=0.3a, whereais an arbitrary reference length. The modulation frequency for the case of panelbisfm=2 × 10−4(c/a). For operation at 1.55 μm, the corresponding absolute values area=1.04 μm,R=0.92 μm,w=0.21 μm andfm=60 GHz. Figure 4: Angular momentum-biased optical isolator based on a channel-drop filter. ( a ) Reciprocal transmission versus frequency of a conventional channel-drop filter. Waves entering from ports 1 and 2 couple to the right- and left-handed resonances of the ring, as illustrated in the left and right insets, respectively, creating a transmission dip at the ring resonance. ( b ) Non-reciprocal transmission versus frequency when spatiotemporal modulation is applied to the ring. The insets show the electric field amplitude distribution at the frequency indicated by the dashed line for excitation from port 1 (left) or 2 (right). The geometrical parameters of the structure are R =0.88 a , w =0.2 a and g =0.3 a , where a is an arbitrary reference length. The modulation frequency for the case of panel b is f m =2 × 10 −4 ( c / a ). For operation at 1.55 μm, the corresponding absolute values are a =1.04 μm, R =0.92 μm, w =0.21 μm and f m =60 GHz. Full size image The simulated scattering parameters of the structure without and with modulation are presented in Fig. 4a,b , respectively. In the absence of modulation, S 21 = S 12 ( S ij being the transmission coefficient from port j to port i ), indicating that the system is reciprocal. When the modulation is applied, the right- and left-handed resonances of the ring split and non-reciprocity occurs, as shown in Fig. 4b . For instance, at the right-handed resonance, indicated in Fig. 4b with the dashed line, transmission from port 1 to 2 is significantly lower than transmission from port 2 to 1, an effect that can also be seen in the corresponding field plots in the inset. This operation is obtained within a ring structure that is comparable in size to the operation wavelength λ =1.55 μm, and without the need of magnetic bias. A new approach to achieve magnetic-free non-reciprocity via angular momentum biasing was presented here on the basis of resonant rings with specifically tailored spatiotemporal azimuthal modulation. The proposed form of modulation removes the degeneracy between opposite resonant states, which, combined with suitably induced high- Q response, realizes giant non-reciprocity in subwavelength components with moderate modulation frequencies and amplitudes. A few applications based on this approach have been presented, including an ultrathin radio frequency isolator, giant Faraday rotation and an optical isolator, all realized without requiring bulky magnetic biasing elements. The proposed approach opens pathways towards many non-reciprocal integrated microwave and nanophotonic components, without requiring magnetic bias, for a variety of applications. Coupled-mode equations neglecting loss and excitation The starting point of our analysis is the coupled-mode theory from Winn et al . [22] for a resonator with a small permittivity perturbation Δ ε ( r , t ). In particular, if a k , ω k and E k are the amplitude, the eigenfrequency and the electric field of the k th mode, where is the coupling coefficient between the k th and th modes. The modes are normalized as where H k is the magnetic field of the k th mode. Noticing that the integral in equation (6) is essentially the energy of the k th mode and that the electric and magnetic energies of a resonator are equal, The eigenspectrum of the ring of Fig. 1a consists of pairs of counter-propagating modes |± k with electric fields where E t k is the electric field of the k th pair in the transverse ρ − z plane. Substituting equation (8) into equation (7), we arrive at the following normalization condition for E t k where S t is the ring cross section. For a permittivity modulation Δ ε ( r , t )=Δ ε m cos ( ω m t −2 φ ) with ω m << ω 1 , the coupling between the |±1 modes and the higher-order modes can be neglected and the coupled-mode equations (4) and (5) reduce to equations (1) and (2). Dividing equations (2) and (9) yields If the modulation is applied to a region, which concentrates most of the field and where ε varies very little, κ m =Δ ε m /(2 ε ). Coupled-mode equations including loss and excitation In the presence of loss, described via a relaxation time τ , the − iω 1 term multiplying a 1 in equation (1) should be substituted by − i ω 1 − τ −1 (ref. 28 ). In addition, when excitation is taken into account the terms − iμ +1 s +1 and − iμ −1 s −1 should be added to the right-hand side of equation (1), where s +1 and s −1 are the components of the incident wave that couple to the |+1 and |−1 states, respectively, and μ +1 and μ −1 are the corresponding coupling coefficients, which are generally functions of the geometry. Then, the coupled-mode equations read These equations support a family of solutions similar to those of equation (3). Discrete capacitance modulation The ring of Fig. 2a is best analysed in terms of voltage V and current I instead of the electric and magnetic fields E and H . Then, the coupled-mode equations (4) and (5) are expected to be valid under the substitutions E → V , H → I , ε → C and μ 0 → L , so that the coupling coefficient is given by where V k = V k 0 e ikφ is the voltage of the k th mode, with V k 0 an appropriate normalization coefficient. For the discretely modulated ring, Then, the coupling coefficients between the −1 and +1 states read If the modulation was continuous, Δ C =Δ C m cos ( ω m t −2 φ ) and Comparing equation (14) with equation (15), we conclude that the discrete modulation is equivalent to a continuous one with amplitude 4Δ C m / π . Full-wave simulations All the numerical simulations of the varactor-loaded ring were performed in the frequency domain by combining a full-wave finite-element electromagnetic simulation (CST Microwave Studio) with a harmonic balance circuit simulation (Agilent Advanced Design System). The numerical domain was terminated with unit cell boundary conditions along the x and y directions and with wave ports along the z direction. The wave ports were used to excite the incident wave and absorb the reflected and transmitted waves. Further, lumped ports were inserted where the variable capacitors were supposed to be connected. The S -parameters obtained through the electromagnetic simulations were imported into the circuit simulator. Ideal variable capacitors, implemented in Agilent Advanced Design System via equation-based non-linear components as shown in the Supplementary Fig. S1 , were connected to the lumped ports of the electromagnetic model and the structure was solved for the S -parameters at the wave ports. The optical ring of Fig. 4 was simulated with a home-made finite-difference time-domain code, where the time-domain permittivity modulation was realized by continuously changing the permittivity of the structure at each time step. The computational domain was terminated with perfectly matched absorbing layers. How to cite this article: Sounas, D.L. et al . Giant non-reciprocity at the subwavelength scale using angular momentum-biased metamaterials. Nat. Commun. 4:2407 doi: 10.1038/ncomms3407 (2013).